Cooperativity and equilibrium with FOXA1 define the androgen receptor transcriptional program The pioneering factor FOXA1 opens chromatin to facilitate androgen receptor (AR) binding to prostate-specific genes. How FOXA1 controls the AR cistrome, however, is incompletely understood. Here we show that AR directly binds chromatin through the androgen response elements (AREs). FOXA1 is not required for AR–chromatin interaction, but instrumental in recruiting AR to low-affinity half-AREs by opening local chromatin around adjacent FKHD sites. Too much FOXA1 creates excessive open chromatin regions, which serve as reservoirs that retain AR via abundant half-AREs, thereby reducing its availability for specific sites. FOXA1 downregulation, by contrast, relinquishes AR to permissively bind AREs across the genome, resulting in substantial AR-binding events and AR target gene expression even in the absence of androgen. Taken together, our data illustrate the mechanistic details by which cooperativity and equilibrium with FOXA1 define AR cistrome and reveal a previously unknown function of FOXA1 in inhibiting AR signalling and castration-resistant prostate cancer growth. The androgen receptor (AR), a hormone-activated transcription factor of the nuclear receptor family, is a key regulator of prostatic gene expression [1] , [2] and plays pivotal roles in prostate differentiation and function [3] . Aberrant elevation of AR signalling, on the other hand, is a critical driver of malignant transformation of the prostate gland and as such androgen-deprivation therapy has been a mainstay treatment of prostate cancer (PCa) [4] . Moreover, AR continues to be upregulated in advanced PCa and its expression and activity remain required for the growth of castration-resistant PCa (CRPC) in an androgen-depleted environment [5] . Studies have shown that AR can become transactivated in CRPC by a number of different mechanisms including AR amplification, AR mutation and alterations in cofactor proteins [6] . AR is a DNA-binding protein that, upon androgen stimulation, binds cis-regulatory elements that harbour the androgen response element (ARE). In addition, like other hormonal receptors such as estrogen receptor, AR often binds distal enhancers, rather than promoters, and regulates target genes through chromatin looping [7] . In order to enable efficient targeting of the AR pathway, numerous studies have attempted to determine the downstream molecules of AR transcriptional regulation. Coupling chromatin immunoprecipitation with next-generation sequencing (ChIP-seq), we and others have revealed tens of thousands of AR-binding events across the human genome at high resolution [8] , [9] . Motif analyses confirmed ARE as the most prevalent DNA motif within AR-binding sites (ARBS), supporting its essential role in mediating AR–DNA interaction. Previous studies have shown that AR–DNA-binding profile is also tightly regulated by an extensive list of cofactors, one key member of which is FOXA1. FOXA1, also known as HNF-3, is a forkhead family transcriptional factor. Possessing winged-helix DNA-binding domains similar to linker histones, FOXA1 is able to access compact chromatin to form high-affinity DNA binding with the FKHD motif and subsequently acts to open up the local nucleosomal domain [10] . FOXA1 is highly expressed in prostate epithelial cells and is critical for the regulation of prostate ductal morphogenesis and epithelial cell differentiation and maturation [11] . This function is largely mediated by the ability of FOXA1 to tightly control AR-modulated transcriptional regulation of prostatic genes [12] . FOXA1 was shown to induce the expression of AR target genes such as PSA by co-occupying the FKHD motif that locates immediately adjacent to the AR-bound ARE motif within the PSA enhancer. Gao et al. [12] have also shown that the FOXA1 protein physically interacts with the AR protein, thereby acting as an AR-collaborating cofactor. Specifically, the DNA-binding domain/hinge region of AR directly interacts with the forkhead domain of FOXA1 (refs 12 , 13 ). Genome-wide location analyses comparing FOXA1-bound genomic regions in prostate and breast cancer cells have revealed cell type-specific recruitment, which subsequently dictates distinct AR and estrogen receptor chromatin-binding patterns in prostate and breast cells, respectively [14] . This model is strongly supported by the findings that FOXA1 binds DNA even in the absence of androgen and preoccupies a majority of the ARBS stimulated by androgen [14] , [15] , [16] . This is especially appealing as FOXA1 is known to act as a pioneer factor that opens up compact chromatin to facilitate the recruitment of other transcription factors including hormonal receptors [10] , [17] , [18] , [19] . Cumulatively, FOXA1 is thus known as a pioneer factor for AR. However, FOXA1 binds substantially more genomic regions than AR and that a majority of FOXA1-binding sites (FXBS) are not co-occupied by AR, arguing that FOXA1 is not sufficient to recruit AR [14] , [15] , [16] . In addition, genome-wide analysis of AR-binding profiles showed that FOXA1 knockdown (KD) resulted in a drastic shift, rather than loss, of ARBS, suggesting that FOXA1 is also not required for AR–chromatin interaction [15] , [16] . How FOXA1 regulates AR cistrome is not fully understood. Here we present evidence that FOXA1 overall inhibits AR signalling, which is mediated by two mechanisms: (1) FOXA1 reduces AR availability to specific ARE sites by facilitating AR binding to numerous half ARE (hARE) sites located within the proximity of FOXA1-bound FKHD sites, and (2) FOXA1 directly inhibits AR gene expression. We further show that FOXA1-KD results in AR binding, target gene expression and PCa cell growth in the absence of androgen. AR DNA-binding ability is required for chromatin occupancy To determine how FOXA1 defines AR-binding profile, we first conducted FOXA1 KD in LNCaP PCa cells and then performed AR and FOXA1 ChIP-Seq in both control and KD cells ( Supplementary Fig. 1A ). As expected, FXBS were drastically reduced following FOXA1 KD ( Fig. 1a ). In addition, ChIP-Seq-read intensity of the remaining FXBS was also significantly decreased ( Supplementary Fig. 1B ). By contrast, AR binding was substantially shifted from some loci to others, confirming reprogramming ( Fig. 1b ). In addition, we observed an overall increase of total ARBS; while ~30% of the initial ARBS were lost twice as many new ones were gained following the silencing of FOXA1. We categorized all ARBS into three categories: present only in control KD cells (shCtrl-only), only in FOXA1-KD cells (shFOXA1-only) or shared in both. Bioinformatics analysis revealed that the shared ARBS have the strongest ChIP-Seq-read intensity, which was further enhanced upon FOXA1 KD, suggesting that they were initially inhibited by FOXA1 ( Fig. 1c,d , Supplementary Fig. 1C ). Surprisingly, the shCtrl-only ARBS were in general quite weak, indicating that FOXA1-dependent AR binding is likely mediated by low-affinity chromatin interactions. By contrast, shFOXA1-only ARBS were of much stronger binding intensity, thus revealing a FOXA1-independent, high-affinity, AR–DNA interaction mechanism. These global patterns were further confirmed through ChIP–qPCR analysis of a representative set of loci from each category ( Supplementary Fig. 1D ) and also in independent replicate experiments ( Supplementary Fig. 2A–D ). 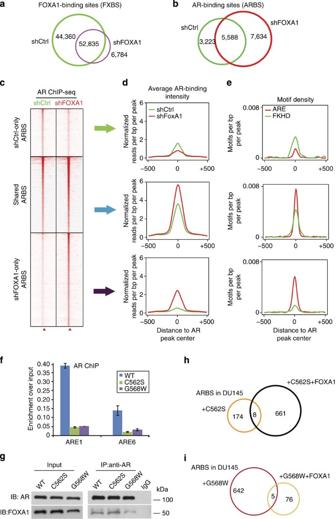Figure 1: The DNA-binding ability of AR is required for its occupancy on the chromatin. (a) Overlap of FXBS. ChIP-Seq of AR and FOXA1 were performed in control (shCtrl) and FOXA1-KD (shFOXA1) LNCaP cells. (b) Overlap of ARBS between shCtrl and shFOXA1 LNCaP cells. (c) Heatmap view of AR and FOXA1 ChIP-Seq-read intensity around ARBS (±2 kb) detected in shCtrl and shFOXA1 LNCaP cells. ARBS were separated into shCtrl-only, shared and shFOXA1-only. (d) Average AR ChIP-seq intensity around ARBS (±500 bp) shown inc. (e) ARE and FKHD motif density around ARBS (±500 bp) shown inc. Motif density was determined by HOMER and normalized to that in a control sequence of equal length. (f) AR mutants (C562S and G568W) had substantially lower ability to bind ARE than wt AR. AR ChIP was done in DU145 cells with stable expression of wt or mutant AR. Error bars indicaten=3, mean±s.e.m.,P<0.05 by two-tailed Student’st-test. (g) AR mutants (C562S and G568W) remained capable of interacting with FOXA1. Co-immunoprecipitation was carried out in DU145 cells with stable expression of wt or mutant AR infected with FOXA1-expressing adenovirus for 48 h. (h,i) FOXA1 failed to increase DNA-binding events of mutant AR. Venn diagram shows overlap of ARBS between control- and FOXA1-expressing DU145+AR (C562S or W568W) cells. Figure 1: The DNA-binding ability of AR is required for its occupancy on the chromatin. ( a ) Overlap of FXBS. ChIP-Seq of AR and FOXA1 were performed in control (shCtrl) and FOXA1-KD (shFOXA1) LNCaP cells. ( b ) Overlap of ARBS between shCtrl and shFOXA1 LNCaP cells. ( c ) Heatmap view of AR and FOXA1 ChIP-Seq-read intensity around ARBS (±2 kb) detected in shCtrl and shFOXA1 LNCaP cells. ARBS were separated into shCtrl-only, shared and shFOXA1-only. ( d ) Average AR ChIP-seq intensity around ARBS (±500 bp) shown in c . ( e ) ARE and FKHD motif density around ARBS (±500 bp) shown in c . Motif density was determined by HOMER and normalized to that in a control sequence of equal length. ( f ) AR mutants (C562S and G568W) had substantially lower ability to bind ARE than wt AR. AR ChIP was done in DU145 cells with stable expression of wt or mutant AR. Error bars indicate n =3, mean±s.e.m., P <0.05 by two-tailed Student’s t -test. ( g ) AR mutants (C562S and G568W) remained capable of interacting with FOXA1. Co-immunoprecipitation was carried out in DU145 cells with stable expression of wt or mutant AR infected with FOXA1-expressing adenovirus for 48 h. ( h , i ) FOXA1 failed to increase DNA-binding events of mutant AR. Venn diagram shows overlap of ARBS between control- and FOXA1-expressing DU145+AR (C562S or W568W) cells. Full size image Our data thus strongly suggest a shifted and gained AR programme in PCa cells following the silencing of FOXA1. To examine whether this may be a phenomenon specific to one cell line, we performed FOXA1 KD in LAPC4 cells using the same small hairpin RNA (shRNA) targeting FOXA1 ( Supplementary Fig. 2E,F ). ChIP–qPCR analysis confirmed that FOXA1 KD resulted in drastic increase of AR binding to the chromatin. This finding was further validated using an independent small interfering RNA (siRNA) that transiently silence FOXA1 in LAPC4 cells, thereby excluding any nonspecific off-target effects ( Supplementary Fig. 2G,H ). Similarly, we found AR overexpression could also lead to AR recruitment to the gained ARBS, supporting that they are authentic AR targets ( Supplementary Fig. 2I,J ). In addition, FOXA1 overexpression strongly suppressed these AR-binding events, further supporting its inhibitory role ( Supplementary Fig. 2K–M ). In addition, FOXA1 was also insufficient in recruiting AR to the DNA since a majority of FXBS were not co-occupied by AR ( Supplementary Fig. 3A,B ). Collectively, our data showed that FOXA1 is neither required nor sufficient for AR–chromatin binding. Next, we examined what modulates the strong AR–chromatin interaction observed in shared and shFOXA1-only ARBS. Motif analysis revealed that strong ARBS (shared and shFOXA1-only) were characterized by high (~30%) incidences of full-ARE motif, while only 7% of shCtrl-only ARBS contained an ARE ( Fig. 1e , Supplementary Fig. 4A ). By contrast, ~45% of shCtrl-only ARBS harboured a FKHD motif, much more than the 15% found in other categories, being consistent with their FOXA1-dependent binding. Shared ARBS, not surprisingly, contained high incidence (~30 and 55%, respectively) of both ARE and FKHD motifs, which explains their resistance to FOXA1 KD. Moreover, de novo motif discovery identified a composite motif containing hARE and FKHD, specifically in shCtrl-only ARBS, suggesting that these weak binding events may be mediated by AR binding to hARE sites, which is facilitated by FOXA1-accessing FKHD motif ( Supplementary Fig. 4B ). To test the importance of direct AR–chromatin interaction, we generated AR mutants C562S and G568W that are deficient in DNA binding but remained capable of interacting with the FOXA1 protein ( Fig. 1f,g ). To assess their ability of DNA binding globally, we infected the AR-negative and FOXA1-negative/low DU145 cells with wild-type (wt) and mutant AR to generate stable clones (DU145+AR, DU145+C562S and DU145+G568W). ChIP-Seq analysis detected very few AR-binding events in the mutant-expressing cells, while ~20,000 AR-binding events were detected in cells expressing wt AR ( Supplementary Fig. 5A ). Next, we concomitantly overexpressed FOXA1 in these cells ( Supplementary Fig. 5B ). Remarkably, ChIP-Seq analysis showed that expression of FOXA1, although led to extensive FOXA1 binding to the chromatin as expected, failed to recruit DNA binding-deficient AR mutants to the chromatin ( Fig. 1h,i and Supplementary Fig. 5C ). Therefore, the DNA-binding ability of AR is absolutely required for its occupancy on the chromatin, supporting its direct interaction with hAREs and full AREs, respectively, in shCtrl-only or shFOXA1-only ARBS. FOXA1 reduces AR–chromatin binding To engineer an independent model to further examine how FOXA1 regulates AR-binding profile, we overexpressed AR in the FOXA1-negative DU145 cells to generate stable cell lines (DU145+AR) ( Supplementary Fig. 6A ). ChIP-Seq analysis revealed abundant AR-binding events in these cells, further supporting that FOXA1 is not required for AR to bind the chromatin ( Fig. 2a ). We next generated DU145+AR+FOXA1 cells that express both FOXA1 and AR. Being consistent with the results observed in LNCaP cells, FOXA1 overexpression shifted AR from its original binding sites to the new genomic loci that were now bound by FOXA1 ( Supplementary Fig. 6B,C ), although the specific AR and FOXA1 programs in DU145 cells differed substantially from those in LNCaP cells ( Supplementary Fig. 7 ). However, these newly acquired FOXA1-dependent ARBS (DU145+AR+FOXA1-only) were of remarkably lower binding intensity than those present in DU145+AR cells (shared and DU145+AR-only ARBS) ( Fig. 2b ). Moreover, the binding intensity of the shared ARBS was also decreased, further supporting an overall inhibition of AR–chromatin occupancy by FOXA1 overexpression. Being consistent with our findings in LNCaP cells, motif analysis showed that strong ARBS were mediated by ARE motifs, whereas the weaker FOXA1-dependent ARBS (DU145+AR+FOXA1-only) harboured remarkably more FKHD motifs ( Fig. 2c ). Overall, FOXA1 overexpression drastically shifted AR binding from high-affinity ARE-containing sites to the genomic loci that harbour FKHD motifs ( Supplementary Fig. 8A,B ). Next, we wondered whether excessive amount of FOXA1 might further recruit AR away from high-affinity sites by inducing more FXBS. 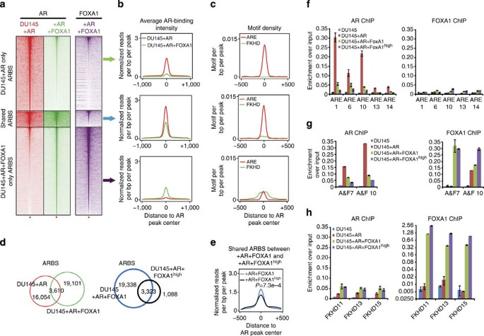Figure 2: FOXA1 reduces AR–chromatin binding. (a) Heatmap view of AR and FOXA1 ChIP-Seq-read intensity around ARBS (±2 kb) that were detected in DU145+AR and DU145+AR+FOXA1 stable cells. ARBS were separated into DU145+AR-only, shared and DU145+AR+FOXA1-only. (b) Average AR ChIP-seq-read intensity around ARBS (±500 bp) shown ina. (c) ARE and FKHD motif density around ARBS (±500 bp) shown ina. Motif density was determined by HOMER and normalized to a control sequence of equal length. (d) Balanced expression of FOXA1 resulted in global redistribution of ARBS, whereas excessive FOXA1 led to remarkable inhibition of ARBS. AR ChIP-Seq was carried out in DU145+AR, DU145+AR+FOXA1 and DU145+AR+FOXA1highcells. The cells were generated by infecting DU145+AR stable cells with LacZ or FOXA1-expressing adenovirus (at 1:2,000 or 1:500 dilution) for 48 h. (e) Average intensity of ARBS shared between DU145+AR+FOXA1 and DU145+AR+FOXA1highcells. (f–h) ChIP–qPCR analysis for AR and FOXA1 occupancy at target regions containing ARE-only (f), ARE and FKHD (A and F) (g) or FKHD-only (h) motifs. ChIP was carried out in DU145+AR, DU145+AR+FOXA1, and DU145+AR+FOXA1highcells. Error bars indicaten=3, mean±s.e.m.,P<0.05 by two-tailed Student’st-test. Figure 2: FOXA1 reduces AR–chromatin binding. ( a ) Heatmap view of AR and FOXA1 ChIP-Seq-read intensity around ARBS (±2 kb) that were detected in DU145+AR and DU145+AR+FOXA1 stable cells. ARBS were separated into DU145+AR-only, shared and DU145+AR+FOXA1-only. ( b ) Average AR ChIP-seq-read intensity around ARBS (±500 bp) shown in a . ( c ) ARE and FKHD motif density around ARBS (±500 bp) shown in a . Motif density was determined by HOMER and normalized to a control sequence of equal length. ( d ) Balanced expression of FOXA1 resulted in global redistribution of ARBS, whereas excessive FOXA1 led to remarkable inhibition of ARBS. AR ChIP-Seq was carried out in DU145+AR, DU145+AR+FOXA1 and DU145+AR+FOXA1 high cells. The cells were generated by infecting DU145+AR stable cells with LacZ or FOXA1-expressing adenovirus (at 1:2,000 or 1:500 dilution) for 48 h. ( e ) Average intensity of ARBS shared between DU145+AR+FOXA1 and DU145+AR+FOXA1 high cells. ( f – h ) ChIP–qPCR analysis for AR and FOXA1 occupancy at target regions containing ARE-only ( f ), ARE and FKHD (A and F) ( g ) or FKHD-only ( h ) motifs. ChIP was carried out in DU145+AR, DU145+AR+FOXA1, and DU145+AR+FOXA1 high cells. Error bars indicate n =3, mean±s.e.m., P <0.05 by two-tailed Student’s t -test. Full size image We engineered DU145+AR cells to express very high amount of FOXA1 ( Supplementary Fig. 6A ). ChIP-Seq analysis confirmed that these cells (DU145+AR+FOXA1 high ) had gained an additional 63,000 FXBS compared with the regular DU145+AR+FOXA1 cells ( Supplementary Fig. 8C ). Surprisingly, there were markedly less AR-binding events in these cells; only 4,400 ARBS were detected compared with the 20,000 ARBS found in DU145+AR or +AR+FOXA1 cells ( Fig. 2d ). With increased FOXA1 expression, nearly 19,000 ARBS were lost with a minimal gain of 1,000 new ones, demonstrating a remarkable effect of FOXA1 in inhibiting AR-binding events. Moreover, even for the conserved ARBS, the read intensity was also substantially reduced ( Fig. 2e and Supplementary Fig. 8D ). Intriguingly, these remaining ARBS were not only co-occupied by FOXA1 but also enriched for strong ARE motifs ( Supplementary Fig. 8E,F ). To validate these important findings, we selected a representative set of genomic loci that contained only ARE, FKHD or both. ChIP–qPCR demonstrated that AR binding to the ARE-only sites was very strong, but drastically reduced following FOXA1 overexpression, and further diminished upon excessive amount of FOXA1 treatment, although these sites were never occupied by FOXA1 ( Fig. 2f ). Similar inhibition, albeit to a lesser extent, was also observed in ARE+FKHD sites, which were co-occupied by FOXA1 as expected ( Fig. 2g ). By contrast, AR binding to FKHD-only sites was in general much weaker, increased upon FOXA1 overexpression, but declined following excessive FOXA1 expression ( Fig. 2h ). Overall, when FOXA1 was overly abundant (in DU145+AR+FOXA1 high cells), AR ChIP-enrichment was very low across all three categories of target regions ( Fig. 2f,h ). Therefore, medium level of FOXA1 shifted AR from high-affinity ARE sites to facilitate their weak binding to FOXA1-bound FKHD sites, while high FOXA1 attenuated all AR-binding events. Next, we attempted to decipher the mechanisms underlying this inhibition. FOXA1 absorbs AR by opening up excessive chromatin regions As FOXA1 has been previously shown to open up compact chromatin to facilitate the access of other transcription factors including AR [14] , we carried out formaldehyde-assisted isolation of regulatory elements (FAIRE)-seq experiments to assay open chromatin regions. Bioinformatics analysis demonstrated that FOXA1 overexpression not only led to a shift but also a great increase in the number of total open chromatin regions ( Fig. 3a ). In addition, a substantial proportion of these open chromatin regions were occupied by FOXA1, confirming the role of FOXA1 as a chromatin-opening factor ( Supplementary Fig. 9A ). To determine how this change in open chromatin relates to the alteration in AR-binding profile, we examined FAIRE-seq signal around ARBS and found that the gained ARBS (DU145+AR+FOXA1-only) indeed became much more accessible following FOXA1 overexpression ( Fig. 3b and Supplementary Fig. 9B ). By contrast, the DU145+AR-only ARBS had drastically reduced chromatin accessibility, which may be due to the loss of AR binding. Interestingly, the FAIRE-seq signal around the shared ARBS remained unaltered, indicating that other mechanisms, such as decreased availability of AR, may be accountable for the attenuation of AR binding around these sites. To validate these global observations, we carried out FAIRE–qPCR and confirmed that, while ARE-only loci became less accessible following FOXA1 overexpression, FKHD-only loci showed dramatically increased accessibility that became several magnitudes higher than the ARE-only sites ( Fig. 3c–e ). The ARE+FKHD sites, on the other hand, had the highest accessibility, which remained largely unchanged following FOXA1 overexpression. 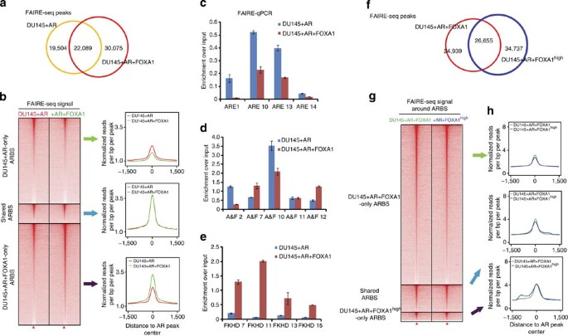Figure 3: FOXA1 opens up chromatin to absorb AR via low-affinity interactions. (a) Overlap between FAIRE-seq peaks identified in DU145+AR and DU145+AR+FOXA1 cells. (b) Heatmap view of FAIRE-seq read intensity around ARBS (5 kb) detected in DU145+AR and/or DU145+AR+FOXA1 stable cells. Shown on the right are average FAIRE-seq counts (±1.5 kb) corresponding to each category of ARBS. (c–e) FAIRE–qPCR analysis of chromatin accessibility at randomly selected loci from ARBS containing ARE-only (c), ARE and FKHD (d) or FKHD-only (e). FAIRE experiment was carried out in DU145+AR and DU145+AR+FOXA1 cells. Overall,P<0.05 for ARE-only sites (c) and FKHD-only sites (e) andPwas not significant on average for all A and F sites (d). Error bars indicaten=3, mean±s.e.m.P-values were calculated by two-tailed Student’st-test. (f) Overlap between FAIRE-seq peaks detected in DU145+AR+FOXA1 and in DU145+AR +FOXA1highcells. (g) Heatmap view of FAIRE-seq read intensity around ARBS (5 kb) detected in DU145+AR+FOXA1 and/or DU145+AR+FOXA1highcells. Shown on the right is average FAIRE-seq signal (±1.5 kb) corresponding to each category of ARBS. Figure 3: FOXA1 opens up chromatin to absorb AR via low-affinity interactions. ( a ) Overlap between FAIRE-seq peaks identified in DU145+AR and DU145+AR+FOXA1 cells. ( b ) Heatmap view of FAIRE-seq read intensity around ARBS (5 kb) detected in DU145+AR and/or DU145+AR+FOXA1 stable cells. Shown on the right are average FAIRE-seq counts (±1.5 kb) corresponding to each category of ARBS. ( c – e ) FAIRE–qPCR analysis of chromatin accessibility at randomly selected loci from ARBS containing ARE-only ( c ), ARE and FKHD ( d ) or FKHD-only ( e ). FAIRE experiment was carried out in DU145+AR and DU145+AR+FOXA1 cells. Overall, P <0.05 for ARE-only sites ( c ) and FKHD-only sites ( e ) and P was not significant on average for all A and F sites ( d ). Error bars indicate n =3, mean±s.e.m. P -values were calculated by two-tailed Student’s t -test. ( f ) Overlap between FAIRE-seq peaks detected in DU145+AR+FOXA1 and in DU145+AR +FOXA1 high cells. ( g ) Heatmap view of FAIRE-seq read intensity around ARBS (5 kb) detected in DU145+AR+FOXA1 and/or DU145+AR+FOXA1 high cells. Shown on the right is average FAIRE-seq signal (±1.5 kb) corresponding to each category of ARBS. Full size image Next, we investigated how excessive FOXA1 results in immense loss of total AR-binding events as illustrated in Fig. 2d,e . FAIRE-seq data showed that high FOXA1 overexpression opened up an additional 10,000 chromatin sites ( Fig. 3f ). This, along with the marvellous gain of FXBS (~63,000), would drastically increase the opportunity for low-affinity AR binding, which was in direct contrast with the observed loss of ~80% of the ARBS. In addition, FAIRE-seq signal around the lost ARBS were only decreased slightly, probably due to increased FOXA1 binding to these sites compensating AR loss ( Fig. 3g ). This eliminates chromatin compacting as a main cause of the loss of ARBS and suggests alternative mechanisms. To determine whether the lost AR still remains on the chromatin, we performed chromatin fractionation followed by immunoblotting, which demonstrated that, in spite of the drastically decreased AR-binding events detected by ChIP-seq, the amount of chromatin-bound AR was surprisingly not reduced by FOXA1 overexpression ( Supplementary Fig. 9C ). These suggest that AR proteins remained on the chromatin but their binding was not detectable by ChIP-Seq. This is plausible as we have previously shown that FXBS-mediated AR-binding events were generally very weak ( Fig. 2a ), which may be further diminished when excessive FOXA1 enables AR to access extensive amount of open chromatin regions. Therefore, FOXA1 opens up chromatin to absorb AR to numerous FXBS via weak interactions, thereby diluting AR and reducing its binding on individual sites. FOXA1 interaction enhances AR binding to ARE+FKHD sites We next asked what mediates the low-affinity AR–chromatin interaction within the FXBS. To address this, we compared the small portion (~10%) of FXBS that were co-occupied by AR with the majority (90%) that were not ( Supplementary Fig. 10A ). FOXA1 ChIP-seq data showed that AR tends to co-occupy relatively strong FXBS, probably due to higher accessibility to these regions ( Supplementary Fig. 10B ). Strikingly, the FXBS that were co-occupied by AR contained much higher occurrence rate of ARE half-sites ( Supplementary Fig. 10C,D ). By contrast, the occurrence of FKHD motif was similar between FXBS with or without AR co-occupancy. Since hARE has substantially less affinity with AR than full ARE, this explains our earlier observation that AR binding to FXBS is generally weaker. Therefore, FOXA1 binding to FKHD sites increases accessibility and facilitates AR binding to the hARE motifs within these sites. As FOXA1 protein has been shown to directly interact with the AR protein [12] , we next asked whether this interaction is required for AR recruitment to the FXBS. We generated an AR mutant (Q640X) that only expresses the AR protein up to position 640, which has been previously shown unable to interact with the FOXA1 protein [12] , [15] . We first confirmed that this mutant was not able to interact with FOXA1 but remained capable of binding ARE-containing DNA ( Fig. 4a and Supplementary Fig. 10E ). In addition, ChIP-Seq analysis of DU145 cells with stable expression of this mutant (DU145+AR_Q640X) demonstrated that it retained the ability to bind the chromatin and a majority of its binding sites overlapped with that of wt AR ( Fig. 4b ). Moreover, FOXA1 overexpression also led to a remarkable shift of the binding profile of the mutant AR, similar to wt AR ( Fig. 4c and Supplementary Fig. 10F ). Most importantly, this shift was also characterized by a dramatic loss of ARE-mediated high-affinity AR-binding events and a substantial gain of FKHD-mediated, FOXA1-dependent weaker ARBS ( Fig. 4d–f ). Together, out data suggest that physical interaction with AR protein is not required for FOXA1 to redistribute AR from ARE to FXBS. These results support that, instead of actively recruiting AR through direct interaction, FOXA1 passively enables AR to access the chromatin. 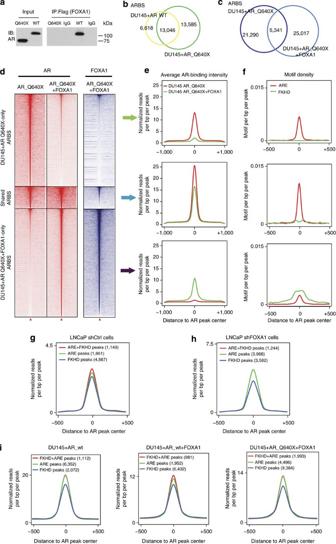Figure 4: FOXA1 and AR protein interaction mediates preferential AR binding to ARE+FKHD sites. (a) Truncated AR (Q640X) failed to interaction with FOXA1. Co-immunoprecipitation experiments were carried out in 293T cells transfected with wt or Q640X-mutant AR along with FOXA1 for 48 h. (b) Overlap of ARBS between DU145+AR (wt) and DU145+AR_Q640X cells. (c) Ectopic expression of FOXA1 resulted in global redistribution of Q640X-mutant AR binding. Venn diagram shows overlap between ARBS detected in DU145+AR_Q640X and in DU145+AR_Q640X+FOXA1 cells. (d) Heatmap view of AR and FOXA1 ChIP-Seq-read intensity around ARBS (±2 kb) detected in DU145+AR_Q640X and in DU145+AR_Q640X+FOXA1 cells. (e) Average AR ChIP-seq intensity around ARBS (±1 kb) shown ind. (f) ARE and FKHD motif density around ARBS (±500 bp) shown ind. (g,h) Average AR ChIP-seq-read intensity around ARBS detected in LNCaP shCtrl cells (g) or in LNCaP shFOXA1 cells (h). Based on the motifs that they contain, ARBS were categorized into ARE+FKHD peaks, ARE-only peaks and FKHD-only peaks. (i) Average AR ChIP-seq-read intensity around ARBS detected in DU145+AR_wt, DU145+AR_wt+FOXA1 or DU145+AR_Q640X+FOXA1 cells. Based on the motifs that they contain, ARBS were separated into ARE+FKHD peaks, ARE-only peaks and FKHD-only peaks. Figure 4: FOXA1 and AR protein interaction mediates preferential AR binding to ARE+FKHD sites. ( a ) Truncated AR (Q640X) failed to interaction with FOXA1. Co-immunoprecipitation experiments were carried out in 293T cells transfected with wt or Q640X-mutant AR along with FOXA1 for 48 h. ( b ) Overlap of ARBS between DU145+AR (wt) and DU145+AR_Q640X cells. ( c ) Ectopic expression of FOXA1 resulted in global redistribution of Q640X-mutant AR binding. Venn diagram shows overlap between ARBS detected in DU145+AR_Q640X and in DU145+AR_Q640X+FOXA1 cells. ( d ) Heatmap view of AR and FOXA1 ChIP-Seq-read intensity around ARBS (±2 kb) detected in DU145+AR_Q640X and in DU145+AR_Q640X+FOXA1 cells. ( e ) Average AR ChIP-seq intensity around ARBS (±1 kb) shown in d . ( f ) ARE and FKHD motif density around ARBS (±500 bp) shown in d . ( g , h ) Average AR ChIP-seq-read intensity around ARBS detected in LNCaP shCtrl cells ( g ) or in LNCaP shFOXA1 cells ( h ). Based on the motifs that they contain, ARBS were categorized into ARE+FKHD peaks, ARE-only peaks and FKHD-only peaks. ( i ) Average AR ChIP-seq-read intensity around ARBS detected in DU145+AR_wt, DU145+AR_wt+FOXA1 or DU145+AR_Q640X+FOXA1 cells. Based on the motifs that they contain, ARBS were separated into ARE+FKHD peaks, ARE-only peaks and FKHD-only peaks. Full size image Next, we examined whether this interaction, although not necessary for AR recruitment, might enhance or stabilize AR binding. We first compared the intensity of endogenous ARBS in LNCaP cells that contain ARE-only, FKHD-only, or both ( Fig. 4g ). Our data confirmed that ARE-mediated binding sites were much stronger than FKHD-mediated ones. In addition, ARBS containing both ARE and FKHD were the strongest, suggesting that FOXA1 co-occupancy in these regions might enhance/stabilize AR binding. Indeed, in FOXA1-KD LNCaP cells, there was no appreciable difference in AR-binding intensity between ARE-only and ARE+FKHD sites, while intensity of both remained superior to that of FKHD-only sites ( Fig. 4h ). To further validate this, we examined ectopically introduced ARBS in DU145 cells. Concordantly, we found that in the absence of FOXA1, the intensity of ARE-only ARBS was the same as those bound to ARE+FKHD sites, both of which were significantly stronger than the FKHD-only sites ( Fig. 4i ). Interestingly, following FOXA1 expression, ARE+FKHD ARBS again became apparently stronger than ARE-only ARBS, which remained superior to the FKHD-only ones. Most importantly, in DU145+AR_Q640X cells wherein FOXA1 was not able to interact with ARE, the preferential AR binding to ARE+FKHD sites was lost. Therefore, physical interaction between FOXA1 and AR enhances AR binding on FKHD+ARE sites, plausibly by locking in both proteins on the chromatin. FOXA1 inhibits AR expression in PCa cells In view of the great increase of ARBS following the silencing of FOXA1 in the endogenous LNCaP system, we asked whether AR might be a direct target of FOXA1-mediated transcriptional repression [20] . We first carried out ChIP–qPCR analysis of the prototype AR target gene KLK3, also called PSA. Our data showed that AR binding to the KLK3 enhancer was indeed drastically increased upon FOXA1 KD ( Fig. 5a ). QRT–PCR analysis further showed that while androgen induced KLK3 expression as expected, FOXA1 KD led to further increase in KLK3 level ( Fig. 5b and Supplementary Fig. 11A ). These increases could be blocked by anti-androgen bicalutamide, supporting the notion that AR transcriptional activity could be augmented upon FOXA1 loss. Analysis of ChIP-seq results indeed revealed a strong FOXA1-binding event within the intragenic region of the AR gene and this binding event was drastically reduced upon FOXA1 KD ( Fig. 5c ). 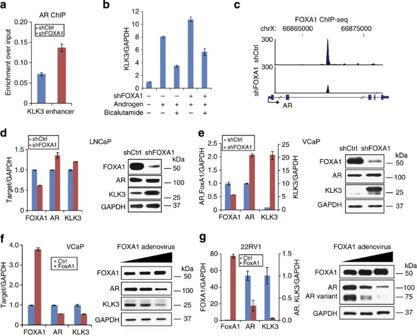Figure 5: FOXA1 inhibits AR gene expression in PCa. (a) AR ChIP was performed in control and shFOXA1 LNCaP cells followed by qPCR analysis of KLK3 enhancer. (b) QRT–PCR analysis of KLK3 expression in control and FOXA1-KD LNCaP cells treated with androgen, anti-androgen bicaluatamide or both. (c) FOXA1 binding to AR intragenic region in LNCaP cell revealed by ChIP-seq. FOXA1 binding is dramatically decreased by FOXA1 KD. (d,e) QRT–PCR and immunoblot analysis of FOXA1, AR and KLK3 in control and FOXA1-KD LNCaP (d) and VCaP cells (e). (f,g) QRT–PCR and immunoblot analysis of FOXA1, AR and KLK3 in VCaP (f) and 22RV1 cells (g) following FOXA1 overexpression. For QRT–PCR, cells were infected with adenovirus (at 1:2,000 dilutions) expressing LacZ control or FOXA1 for 48 h. For immunoblot analysis, cells were infected with increasing amount of FOXA1 adenovirus at 1:8,000, 1:2,000 or 1:500 dilutions. Error bars indicaten=3, mean±s.e.m.,P<0.05 by two-tailed Student’st-test. Figure 5: FOXA1 inhibits AR gene expression in PCa. ( a ) AR ChIP was performed in control and shFOXA1 LNCaP cells followed by qPCR analysis of KLK3 enhancer. ( b ) QRT–PCR analysis of KLK3 expression in control and FOXA1-KD LNCaP cells treated with androgen, anti-androgen bicaluatamide or both. ( c ) FOXA1 binding to AR intragenic region in LNCaP cell revealed by ChIP-seq. FOXA1 binding is dramatically decreased by FOXA1 KD. ( d , e ) QRT–PCR and immunoblot analysis of FOXA1, AR and KLK3 in control and FOXA1-KD LNCaP ( d ) and VCaP cells ( e ). ( f , g ) QRT–PCR and immunoblot analysis of FOXA1, AR and KLK3 in VCaP ( f ) and 22RV1 cells ( g ) following FOXA1 overexpression. For QRT–PCR, cells were infected with adenovirus (at 1:2,000 dilutions) expressing LacZ control or FOXA1 for 48 h. For immunoblot analysis, cells were infected with increasing amount of FOXA1 adenovirus at 1:8,000, 1:2,000 or 1:500 dilutions. Error bars indicate n =3, mean±s.e.m., P <0.05 by two-tailed Student’s t -test. Full size image To determine whether this FOXA1-binding event leads to regulation of AR gene expression, QRT–PCR was carried out and showed that AR and KLK3 expression were indeed significantly increased following FOXA1 KD ( Fig. 5d ). Immunoblotting demonstrated remarkably upregulated KLK3 protein along with a slight increase of the AR protein. Similar results were also observed in other PCa cells including VCaP ( Fig. 5e ) and 22RV1 cells ( Supplementary Fig. 11B ). To preclude off-target shRNA effects, we used an siRNA that targets a different region of the FOXA1 gene and confirmed that FOXA1 KD indeed increased AR and KLK3 expression in PCa cells ( Supplementary Fig. 11C,D ). As western blot revealed only slight increase of AR protein upon FOXA1 KD, probably due to already very high level of AR in control cells, we took an alternative approach to overexpress FOXA1 in these cells to examine AR inhibition. Using FOXA1-expressing adenovirus, we demonstrated that FOXA1 overexpression remarkably suppressed both AR and KLK3 transcript and protein in PCa cells ( Fig. 5f,g ). Taken together, in addition to reducing specific AR binding by absorbing AR to excessive amount of open chromatin, FOXA1 also directly inhibited AR expression. This poses a pathologically important question as to whether FOXA1 loss in advanced PCa, as recently reported by us and others [15] , [20] , might contribute to aberrant AR activation. FOXA1 loss results in androgen-independent AR binding events We first examined whether FOXA1 continues to inhibit AR in the absence of androgen. QRT–PCR and western blot analysis demonstrated that FOXA1 KD in hormone-deprived LNCaP cells increased AR expression and led to significant upregulation of KLK3 transcript as well as protein ( Fig. 6a ). In particular, although western blot was only able to detect slight increase in total AR protein, nuclear AR and chromatin-bound AR were both dramatically increased following the silencing of FOXA1 ( Fig. 6b ). This suggests that loss of FOXA1 activated AR–chromatin binding in the absence of androgen. Indeed, ChIP–qPCR demonstrated remarkably increased AR binding on the KLK3 enhancer at a level comparable with androgen stimulation ( Supplementary Fig. 12A ). Concordantly, the expression levels of both KLK3 transcript and protein were drastically induced, which could be blocked by AR KD ( Fig. 6c,d and Supplementary Fig. 12B ). Most importantly, downregulation of FOXA1 significantly increased androgen-independent cell growth, reflecting the activation of the AR signalling pathway and its pathological relevance ( Fig. 6e ).To determine whether FOXA1 loss activates androgen-independent AR–chromatin binding globally, we mapped the genomic landscape of AR in the control and FOXA1-KD LNCaP cells that were grown in hormone-deprived medium. As expected, there were very few AR-binding events (508 ARBS) in the androgen-depleted control cells. Remarkably, following the silencing of FOXA1, a substantial amount of AR-binding events (over fourfold increase) was detected even in the absence of androgen ( Fig. 6f ). 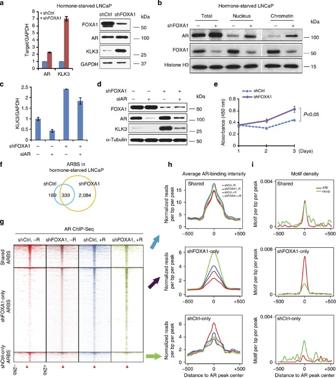Figure 6: FOXA1 downregulation results in AR–chromatin binding in the absence of androgen. (a) QRT–PCR and immunoblot analyses of AR, FOXA1 and KLK3 were performed in hormone-starved control and shFOXA1 LNCaP cells. GAPDH was used as a loading control. Error bars indicaten=3, mean±s.e.m.,P<0.05 by two-tailed Student’st-test. (b) Total lysate, nuclear proteins and chromatin fraction were collected or isolated from hormone-starved control and FOXA1-KD LNCaP cells and western blot was performed with indicated antibodies. (c,d) Control and shFOXA1 LNCaP cells were hormone deprived and subjected to RNA interference targeting control or AR (siAR). KLK3 gene expression was determined by QRT–PCR Error bars indicaten=3, mean±s.e.m.P<0.05 by two-tailed Student’st-test. (c). Protein levels of KLK3, AR and FOXA1 were analysed by immunoblot (d). (e) Silencing of FOXA1 results in androgen-independent cell growth. LNCaP shCtrl and shFOXA1 cells were grown in hormone-deprived, phenol-free RPMI 1640 media supplemented with 5% charcoal-stripped fetal bovine serum. Total cell growth was measured by WST-1 assay as previously reported20. Error bars indicaten=3, mean±s.e.m. SignificantP-value was indicated. (f)AR ChIP-Seq was performed using hormone-deprived control and FOXA1-KD LNCaP cells. Venn diagram shows the overlap of ARBS between these two cell types. (g) Heatmap view of AR ChIP-seq-read density around ARBS (±2 kb). ARBS detected in hormone-deprived shCtrl and shFOXA1 LNCaP cells were separated into shCtrl-only, shared and shFOXA1-only. ‘−R’ indicated androgen-depleted medium, whereas ‘+R’ indicated regular medium for LNCaP cell culture. (h) Average AR ChIP-seq intensity around ARBS (±500 bp) shown inf. (i) ARE and FKHD motif density around ARBS (±500 bp) shown inf. Figure 6: FOXA1 downregulation results in AR–chromatin binding in the absence of androgen. ( a ) QRT–PCR and immunoblot analyses of AR, FOXA1 and KLK3 were performed in hormone-starved control and shFOXA1 LNCaP cells. GAPDH was used as a loading control. Error bars indicate n =3, mean±s.e.m., P <0.05 by two-tailed Student’s t -test. ( b ) Total lysate, nuclear proteins and chromatin fraction were collected or isolated from hormone-starved control and FOXA1-KD LNCaP cells and western blot was performed with indicated antibodies. ( c , d ) Control and shFOXA1 LNCaP cells were hormone deprived and subjected to RNA interference targeting control or AR (siAR). KLK3 gene expression was determined by QRT–PCR Error bars indicate n =3, mean±s.e.m. P <0.05 by two-tailed Student’s t -test. ( c ). Protein levels of KLK3, AR and FOXA1 were analysed by immunoblot ( d ). ( e ) Silencing of FOXA1 results in androgen-independent cell growth. LNCaP shCtrl and shFOXA1 cells were grown in hormone-deprived, phenol-free RPMI 1640 media supplemented with 5% charcoal-stripped fetal bovine serum. Total cell growth was measured by WST-1 assay as previously reported [20] . Error bars indicate n =3, mean±s.e.m. Significant P -value was indicated. ( f )AR ChIP-Seq was performed using hormone-deprived control and FOXA1-KD LNCaP cells. Venn diagram shows the overlap of ARBS between these two cell types. ( g ) Heatmap view of AR ChIP-seq-read density around ARBS (±2 kb). ARBS detected in hormone-deprived shCtrl and shFOXA1 LNCaP cells were separated into shCtrl-only, shared and shFOXA1-only. ‘−R’ indicated androgen-depleted medium, whereas ‘+R’ indicated regular medium for LNCaP cell culture. ( h ) Average AR ChIP-seq intensity around ARBS (±500 bp) shown in f . ( i ) ARE and FKHD motif density around ARBS (±500 bp) shown in f . Full size image We next examined how these androgen-independent ARBS relate to the normal androgen-stimulated AR-binding events. To do this, we categorized these ARBS into control-only, shFOXA1-only and shared, and examined these binding profiles in both androgen-deprived and androgen-stimulated conditions. Heatmap view of ChIP-seq-read intensity confirmed remarkable AR recruitment to the shFOXA1-only sites upon FOXA1 KD, despite a clear loss of FOXA1 binding ( Fig. 6g and Supplementary Fig. 12C ). Moreover, androgen stimulation was also able to recruit AR to these sites and showed a synergistic effect with FOXA1 KD ( Fig. 6h ). These results support that FOXA1 downregulation induces AR binding in the absence of androgen. For example, while a few AR binds the KLK3 enhancer in the control cells before androgen treatment, FOXA1 KD can lead to substantial AR recruitment, which is further enhanced by androgen stimulation ( Supplementary Fig. 12D ). Motif analysis revealed that the ARE motifs were strongly enriched in the ARBS gained upon FOXA1 KD ( Fig. 6i and Supplementary Fig. 4A ). Next, we investigated whether this increase in AR–chromatin binding by FOXA1 KD activates a corresponding AR transcriptional programme in the absence of androgen. FOXA1 loss activates a castration-resistant AR program To determine the AR-mediated transcriptional programme, we carried out microarray analysis of control and FOXA1-KD LNCaP cells grown in androgen-depleted medium. We separated FOXA1-regulated genes into FOXA1-induced and repressed and compared with those induced or repressed by androgen. Interestingly, GSEA analysis revealed that genes induced by FOXA1 in the absence of androgen significantly overlapped with those repressed by androgen, while FOXA1-repressed genes were enriched for androgen-induced genes ( Fig. 7a,b ). Therefore, in the absence of androgen, FOXA1 exhibited a transcriptional regulatory role that antagonizes AR. This is consistent with our ChIP-seq data indicating that FOXA1 KD induces AR–chromatin binding in the absence of androgen. Indeed, GSEA analysis showed that androgen-induced genes on the other hand were enriched for upregulation by FOXA1 KD, while androgen-repressed genes tended to become downregulated following the silencing of FOXA1 in hormone-deprived LNCaP cells ( Fig. 7c,d ). Furthermore, QRT–PCR analysis confirmed that known androgen-induced genes such as KLK3,TMPRSS2, FKBP5 and KLK2 were strongly induced by FOXA1 KD in hormone-deprived LNCaP cells, while previously reported androgen-repressed genes were inhibited ( Figs 6c , 7e,f ), in concordance with gained ARBS on main AR-binding loci of these genes upon FOXA1 depletion ( Supplementary Fig. 13A–E ). Therefore, FOXA1 loss induces AR transcriptional programme. In addition, gene ontology (GO) analysis of shFOXA1-induced gene set ( Supplementary Data 1 ) revealed ‘response to steroid hormone’, ‘regulation of cell proliferation’ and ‘locomotion/cell migration’ as the enriched GO terms ( Supplementary Fig. 14 ). This indicates that FOXA1 loss, like AR overexpression, provides important means to aberrant AR activation in the milieu of very low androgen. 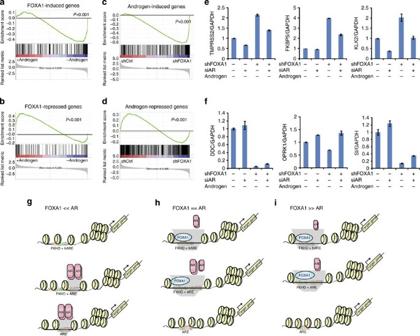Figure 7: FOXA1 loss activates a castration-resistant AR transcriptional programme. (a,b) GSEA was carried out using FOXA1-induced or FOXA1-repressed gene set comparing control and androgen-treated LNCaP cells. Genes induced by FOXA1 in hormone-starved LNCaP cells are enriched for repression by androgen (a). Genes repressed by FOXA1 in hormone-starved LNCaP cells are enriched for induction by androgen (b). FOXA1-induced or repressed gene set (with 2-fd cutoff) was obtained from microarray profiling control and shFOXA1 LNCaP cells grown in hormone-starved condition. Microarray data have been previously released at GEO under accessionGSE37314(ref.20). (c,d) GSEA reveals that androgen-induced genes correlate with higher expression in shFOXA1 cells relative to control cells (c), while androgen-repressed genes are significantly enriched for downregulation in shFOXA1 cells (d). Androgen-induced and -repressed genes were identified from microarrays of LNCaP shCtrl –R cells and LNCaP shCtrl +R cells using a cutoff of ≥twofold change. Expression data set are from microarray profiling of hormone-starved LNCaP shCtrl and shFOXA1 cells as above mentioned. (e,f) QRT–PCR analysis of expression of three typical androgen-induced genes (e) and three androgen-repressed genes (f) in hormone-starved LNCaP cells treated with shFOXA1, siAR or both. All error bars indicaten=3, mean±s.e.m. (g–i) Model of FOXA1 regulation of AR–chromatin binding in a dose- and context-dependent manner. (g) When FOXA1 is relative low or absent, AR is freely available to bind genomic regions containing ARE. (h) When FOXA1 and AR levels are in equilibrium, FOXA1 opens up FKDH-containing chromatin regions to facilitate AR binding to these sites, thereby preventing AR binding to ARE-only sites. (i) When FOXA1 is much more abundant than AR, it opens up excessive amount of chromatin regions, which end up diluting AR across the genome, thereby inhibiting specific AR-binding events. Cup-shape shaded areas indicate chromatin accessibility. hARE indicates low-affinity ARBS with hARE motif, compared with high-affinity ARBS with canonical ARE motif. Figure 7: FOXA1 loss activates a castration-resistant AR transcriptional programme. ( a , b ) GSEA was carried out using FOXA1-induced or FOXA1-repressed gene set comparing control and androgen-treated LNCaP cells. Genes induced by FOXA1 in hormone-starved LNCaP cells are enriched for repression by androgen ( a ). Genes repressed by FOXA1 in hormone-starved LNCaP cells are enriched for induction by androgen ( b ). FOXA1-induced or repressed gene set (with 2-fd cutoff) was obtained from microarray profiling control and shFOXA1 LNCaP cells grown in hormone-starved condition. Microarray data have been previously released at GEO under accession GSE37314 (ref. 20 ). ( c , d ) GSEA reveals that androgen-induced genes correlate with higher expression in shFOXA1 cells relative to control cells ( c ), while androgen-repressed genes are significantly enriched for downregulation in shFOXA1 cells ( d ). Androgen-induced and -repressed genes were identified from microarrays of LNCaP shCtrl –R cells and LNCaP shCtrl +R cells using a cutoff of ≥twofold change. Expression data set are from microarray profiling of hormone-starved LNCaP shCtrl and shFOXA1 cells as above mentioned. ( e , f ) QRT–PCR analysis of expression of three typical androgen-induced genes ( e ) and three androgen-repressed genes ( f ) in hormone-starved LNCaP cells treated with shFOXA1, siAR or both. All error bars indicate n =3, mean±s.e.m. ( g – i ) Model of FOXA1 regulation of AR–chromatin binding in a dose- and context-dependent manner. ( g ) When FOXA1 is relative low or absent, AR is freely available to bind genomic regions containing ARE. ( h ) When FOXA1 and AR levels are in equilibrium, FOXA1 opens up FKDH-containing chromatin regions to facilitate AR binding to these sites, thereby preventing AR binding to ARE-only sites. ( i ) When FOXA1 is much more abundant than AR, it opens up excessive amount of chromatin regions, which end up diluting AR across the genome, thereby inhibiting specific AR-binding events. Cup-shape shaded areas indicate chromatin accessibility. hARE indicates low-affinity ARBS with hARE motif, compared with high-affinity ARBS with canonical ARE motif. Full size image Previous studies have established a model wherein FOXA1 protein acts as a pioneering factor that interacts with and recruits AR to lineage-specific binding sites [14] . Interestingly, two studies recently reported that FOXA1 KD resulted in extensive AR reprogramming rather than elimination, suggesting that FOXA1 may be pioneering for AR binding to some sites but inhibitory to other sites [15] , [16] . The mechanisms underlying this reprogramming, however, were not well understood. In the present study, we reconcile these conflicting results by providing a refined model wherein FOXA1 controls the genomic landscape of AR by altering chromatin accessibility, which may result in cooperative or inhibitory effects on AR programme depending on the relative FOXA1/AR abundance ( Fig. 7g–i ). FOXA1 is neither required nor sufficient to recruit AR binding. Rather, FOXA1 opens up chromatin to preferentially facilitate AR to access FOXA1-bound genomic regions. When AR is much more abundant than FOXA1 (for example, in LNCaP+shFOXA1 or DU145+AR cells), AR primarily binds to its high-affinity target ARE sites across the genome ( Fig. 7g ). When FOXA1 reaches equilibrium with AR (for example, LNCaP cells), FOXA1 opens up FKHD-containing regions to permit AR interaction with either low-affinity hAREs or high-affinity full-AREs that are located within these regions, manifesting a collaborative role ( Fig. 7h ). This, however, is accomplished by removing AR from high-affinity ARE sites located outside of FXBS, as illustrated by the extensive loss of ARE-only ARBS. When FOXA1 becomes overly abundant (for example, hormone-deprived LNCaP cells or DU145+AR+FOXA1 high cells), FOXA1 opens up excessive amount of genomic regions, which act as a reservoir that absorbs AR through low-affinity interactions and thus drastically reduces the amount of AR available for any individual loci. In this condition, FOXA1 inhibits almost all specific AR–chromatin binding ( Fig. 7i ). This context-dependent regulation may be critical in offsetting androgen response in hormone-deprived condition and in maximizing rapid response upon androgen stimulation, which should be carefully examined in future studies. Our proposed model demonstrates multifaceted roles of FOXA1 in tightly controlling AR signalling and provides mechanisms that reconcile previously reported roles of FOXA1 as an AR-collaborating or inhibiting co-factor [14] , [15] , [16] . Importantly, we believe that our model precisely recapitulates how FOXA1 dictates prostatic-specific gene expression. Had FOXA1 not affected AR–chromatin binding, AR would have been relinquished to bind ARE motifs across the genome, which are not specific to prostate genes. On the other hand, had FOXA1 directly recruited AR to the genome AR would potentially get recruited to all FXBS, which would ultimately dilute AR and inhibits AR-mediated activation of prostate-specific genes. Our model, by contrast, showed that when FOXA1 is in equilibrium with AR, it opens up the chromatin to preferably facilitate AR co-occupancy at FKHD+ARE sites (high-affinity and highly accessible), but reduces AR binding to ARE-only sites (high affinity but not accessible). Therefore, our study not only supports previously reported roles of FOXA1 in specifying lineage-specific AR programme [14] , but also delineates the mechanistic details of this regulation. The ability of FOXA1 to inhibit high-affinity ARE-mediated AR–chromatin binding is not only essential in defining a prostatic AR programme but also critical in preventing non-prostatic AR-binding events. Recent studies have shown that such programme could be highly oncogenic [15] and alteration of this regulatory pathway may turn on novel AR target genes in CRPC [21] . Future studies should examine how the balanced regulation between FOXA1 and AR is disrupted during PCa progression. In this study, we have also shown that FOXA1 directly inhibits AR expression and thus the transcription of its target genes. Interestingly, consistent with our results, a recent study has shown that FOXA1 overexpression largely inhibits AR target genes in PCa cells [22] and decreases cell motility and tumour metastasis [15] , [20] . Most importantly, our study revealed that FOXA1 loss activates AR–chromatin binding and AR transcriptional regulation in the absence of androgen. This activation may be due to the fact that FOXA1 KD enabled the cells to reach a new balance between reduced FOXA1 and the low amount of nuclear AR available in hormone-deprived cells, thereby permitting high-affinity AR binding. In addition, cell growth assay showed increased PCa cell growth following the silencing of FOXA1 in androgen-depleted medium. These findings suggest that loss of FOXA1 may lead to androgen-independent AR signalling and thus CRPC progression. Indeed, we have recently reported that FOXA1 is downregulated in CRPC [20] . Due to the multifaceted roles of FOXA1 in regulating AR signalling that is heavily dependent on FOXA1-AR equilibrium, the pathological relevance of FOXA1 may be elusive. In fact, there are apparent conflicting reports that linked FOXA1 expression levels with either good or bad clinical outcomes. Based on our model, it is possible that FOXA1 may be associated with poor prognosis if the analysis is solely based on patients with primary PCa [16] or metastatic PCa [23] who have not received prior systematic therapy. However, FOXA1 may be a good outcome predictor in patient cohorts with prior androgen-deprivation therapy [15] . It is thus very important to re-evaluate FOXA1 association with PCa outcomes in future studies by carefully stratifying patients based on their disease stage and treatment histories. Taken together, our study delineates the mechanism by which FOXA1 defines the genomic action of AR and provides a novel pathway to aberrant AR activation in the milieu of very low androgen. Cell Culture and antibodies LNCaP, DU145, 22RV1 and VCaP cells were obtained from the American Type Culture Collection (ATCC) and grown in RPMI or DMEM (VCaP) supplemented with 10% fetal bovine serum and standard antibiotics. LAPC4 cells were provided by Dr C Shad Thaxton (Northwestern University) and grown in IMEM supplemented with 10% fetal bovine serum and 1 nm R1881. For androgen treatment, cells were hormone starved for 2–3 days and treated with 1 nM R1881 for 24 h. Bicalutamide (Casodex) was added at a concentration of 10 μM as needed. Antibodies used in this study include anti-AR (06-680) from Millipore, anti-FOXA1 (ab23738), Histone H3 (ab1791) and anti-GAPDH (ab9385) from Abcam, anti-AR (sc-7305) from Santa Cruz and anti-KLK3 (K2889-100UG) from Sigma ( Supplementary Table 3 ). siRNA, shRNA and Plasmids FOXA1 siRNA (sense 5′-GAGAGAAAAAAUCAACAGC-3′; antisense 5′-GCUGUUGAUUUUUUCUCUC-3′) [14] , [20] , AR on-target plus smart pool (L-003400-00-0020), and control siRNA Luciferase GL2 Duplex (D-001100-01-20) were synthesized by Dharmacon. The control and pGIPZ lentiviral shRNAmir targeting FOXA1 (Clone ID# V2LHS_16780) were purchased from Open Biosystems. C-terminal 3 × HA-tagged full-length FOXA1 was cloned into a Tet-On inducible lentiviral vector that was kindly provided by Professor Junjie Chen (MD Anderson Cancer Center). The full-length (wt) and truncated AR (Q640X) were amplified from pcDNA3.1-AR fl plasmid [24] and cloned into the pCR8/GW/TOPO entry vector (Invitrogen). The pCR8-AR C562S and G568W mutants were generated from pCR8-AR wt using QuikChange II Site-Directed Mutagenesis Kit (Agilent Technologies, Santa Clara, CA). Lentiviral constructs were generated by LR recombination between pCR8-AR constructs and pLenti CMV/TO Puro DEST (Addgene plasmid 17293). Details regarding cloning primers and plasmid construction were provided in Supplementary Tables 1 and 2 . Western blot analysis Cells were lysed in NP40 Cell Lysis Buffer (Invitrogen). Protein concentration was measured using the Bio-Rad protein assay kit. Twenty micrograms of the total protein were mixed with SDS sample buffer, boiled for 10 min at 95 °C, separated on a 10% SDS-polyacrylamide gel and transferred to an Amersham Hybond PVDF membrane. The membranes were blocked with 5% w/v BSA or milk in TBST overnight at 4 °C, incubated in primary antibody (diluted in blocking solution) for either 1 h at room temperature or overnight at 4 °C (for antibodies, see Supplementary Table 3 ), washed 3 × with TBST and incubated for 1 h in a secondary antibody diluted in blocking solution. Membranes were again washed 3 × with TBST and ECL (GE Healthcare) was added to the membrane and the signal was detected on film (GE Healthcare). Representative uncropped raw scans of blots generated with the most relevant antibodies used along the different figures are present in Supplementary Figs 15–17 . Co-immunoprecipitation Cells with coexpression of FOXA1 (tagged with Flag) and AR (wt or mutant) were lysed in IP lysis buffer (50 mM Tris-Cl pH7.4, 150 mM NaCl, 1 mM EDTA, 1% Triton X-100, Roche protease inhibitor cocktail). An aliquot of the cell lysate was kept as input for western blot analysis. Cell lysate was first precleared with protein A/G-agarose beads at 4 °C for 2 h. Then the precleared lysate was incubated with mouse anti-Flag (F1804, Sigma) or mouse anti-AR antibody (sc-7305, Santa Cruz), mouse IgG (as a negative control) overnight on a rocker platform. The next day, protein A/G-agarose beads were added to the mixture and incubated at 4 °C for 2 h. Then the beads were pelleted and washed for four times with IP lysis buffer before boiling in SDS sample buffer for 10 min. Western blotting analysis were performed using rabbit anti-FOXA1(ab23738, Abcam) or rabbit anti-AR(06-680, Millipore). Chromatin fractionation Chromatin was isolated as described with the following modifications [25] . Cells were resuspended in buffer A (10 mM HEPES, [pH 7.9], 10 mM KCl, 1.5 mM MgCl2, 0.34 M sucrose, 10% glycerol, 1 mM DTT, 1 × Roche protease inhibitor cocktail). Triton X-100 (0.1%) was added, and the cells were incubated for 5 min on ice. Nuclei were collected in pellet 1 by low-speed centrifugation (5 min, 1,300 g , 4 °C), washed once with buffer A, and then resuspended in buffer B (3 mM EDTA, 0.2 mM EGTA, 1 mM DTT, protease cocktail) for 30 minutes on ice. Insoluble chromatin was isolated by centrifugation (5 min, 1,700 g , 4 °C), washed once with buffer B, and centrifuged again under the same conditions. The final chromatin pellet was resuspended in SDS sample buffer (50 mM Tris-HCl pH 6.8, 2% SDS, 10% glycerol, 2% β-mercaptoethanol and 0.02% bromophenol blue). Chromatin immunoprecipitation (ChIP) AR and FOXA1 ChIP were carried out as described previously [9] , [26] , [27] . Briefly, cultured cells were cross-linked with 1% formaldehyde for 10 min and the cross-linking was inactivated by 0.125 M glycine for 5 min at room temperature. Cells were then rinsed with cold 1 × PBS twice. The following steps were performed at 4 °C. Cell pellets were resuspended and incubated in cell lysis buffer+10 ul ml −1 PMSF and protease inhibitor (Roche) for 10 min. Nuclei pellets were spinned down at 5,000 g for 5 min, resuspended in nuclear lysis buffer and then incubated for another 10 min. Chromatin was sonicated to an average length of 500 bp and then centrifuged at 14,000 g for 10 min to remove the debris. Supernatants containing chromatin fragments were incubated with agarose/protein A or G beads (Upstate) for 15 min and centrifuged at 5,000 g for 5 min to reduce nonspecific binding. To immunoprecipitate protein/chromatin complexes, the supernatants were incubated with 3–5 ug of antibody (anti-FOXA1 from Abcam, cat# ab23738; anti-AR from Millipore, cat#06-680) overnight, then added 50 ul of agarose/protein A or G beads and incubated for 1.5 h. Beads were washed twice with 1X dialysis buffer and four times with IP wash buffer. The antibody /protein/DNA complexes were eluted with 150 ul IP elution buffer twice. To reverse the cross-links, the complexes were incubated in elution buffer+10 ug RNase A and 0.3 M NaCl at 67 °C for 4 h. DNA/proteins were precipitated with ethanol, air-dried and dissolved in 100 ul of TE. Proteins were then digested by proteinase K at 45 °C for 1 h and DNA was purified with QIAGEN PCR column and eluted with 30 ul EB. Formaldehyde-assisted isolation of regulatory elements FAIRE was performed according to the protocol published by Giresi et al. [28] Briefly, cells were cross-linked identically as for ChIP. After 10-min cross-linking with 1% formaldehyde and stopping with 0.125 M glycine, the washed cell pellets (10 e7 cells) were resuspended and incubated for 10 min sequentially in 1 ml of buffer L1, 1 ml of buffer L2 and 400 μl of buffer L3. The lysates were sonicated in order to shear chromatin into DNA fragments of average 300–500 bp, then centrifuged at 14,000 g for 10 min to remove the cellular debris. Input samples were reverse cross-linked overnight at 65 °C. The FAIRE samples and reverse cross-linked input samples were subjected to three sequential phenol/chloroform/isoamyl alcohol (25/24/1) extractions. DNA were precipitated with ethanol, air-dried and dissolved in 100 ul of TE and treated with 1 μl of RNase A (10 mg ml −1 ) for 1 h at 37 °C. Proteins were then digested by proteinase K at 45 °C for 1 h and the DNA was purified with QIAquick PCR Purification Kit (Qiagen) and eluted with 30 ul EB. Quantitative Polymerase Chain Reaction All primers ( Supplementary Table 1 ) were designed using Primer 3 ( http://frodo.wi.mit.edu/primer3/ ), and synthesized by Integrated DNA Technologies. SYBR Green based quantitative real-time PCR was performed using GoTaq qPCR MasterMix (Promega) using a StepOnePlus Real-Time PCR System (Applied Biosystems). For quantitative reverse transcription-PCR (QRT–PCR) data analysis, the fold change in the target gene relative to the GAPDH (glyceraldehyde 3-phosphate dehydrogenase) endogenous control gene is determined by: fold change=2 –Δ(ΔCt) where ΔCt=Ct target –Ct GAPDH and Δ(ΔCt)=ΔCt treatment –ΔCt control . For ChIP–qPCR and FAIRE–qPCR, enrichment analysis were performed by Comparative Ct method and normalization to input, that is, enrichment over input=2 (–ΔCt) , where ΔCt=Ct sample −Ct input . ChIP-seq and FAIRE-seq library preparation and sequencing Libraries were prepared according to standard protocols using BioScientific’s DNA Sample Kit (Cat# 514101) [9] , [27] . Libraries were sequenced using Illumina Hi-Seq platforms. Sequence reads were aligned to the Human Reference Genome (assembly hg19) using Burrows-Wheeler Alignment (BWA) Tool version 0.6.1 (ref. 29 ). ChIP-seq and FAIRE-seq peak discovery ChIP-seq and FAIRE-seq peak identification, overlap, subtraction, union and feature annotation of enriched regions were performed using HOMER (Hypergeometric Optimization of Motif EnRichment) suite ( http://homer.salk.edu/homer/ ) [30] . For ChIP-seq, HOMER peak finding algorithm searches for peaks of fixed size to achieve maximum sensitivity. For FAIRE-seq analysis, we used HOMER to find variable-width enriched regions. Homer automatically optimized parameters needed for peak finding the size of the peak and the length of fragments. We set the minimum distance between peaks using 2.5 × the peak size. The cutoff for statistically significant peaks was selected at a false discovery rate of 0.001 determined by peak finding using randomized tag positions in a genome with an effective size of 2 billion basepairs. We required the tag density at peaks to be fourfold greater than in the surrounding 10 kb region to exclude putative peaks identified in regions of genomic duplication. Only one tag from each unique position was considered to filter clonal signal from the sequencing. Additional peak calls were determined using MACS peak caller version 1.4.1 (ref. 31 ) with default parameters, in which enriched regions of the genome were identified by comparing the ChIP samples to input samples. The number of sequencing reads and AR or FOXA1-binding events for each sample were shown in Supplementary Table 4 . Motif discovery The HOMER motif discovery was used to perform de novo motif discovery as well as check the enrichment of known motifs in a set of given genomic region (200 bp surrounding ChIP-seq peak center) [30] . Motif density histograms were created using HOMER for target regions. Control regions were generated by selecting DNA sequences of equal length at 10 kb downstream of the target regions. The motif density at target regions was normalized to that at the control regions. Additional motif analysis was determined using MEME-ChIP algorithm [32] . Gene expression array and data analysis Total RNAs were isolated using TRIzol reagent (Invitrogen). The integrity of the RNA was monitored using Bioanalyzer 2100. Microarray profiling was performed using HumanHT-12 v 4.0 Expression BeadChip (Illumina). Bead-level data were preprocessed using GenomeStudio (Illumina), and the expression values were quantile-normalized using the bead array package in Bioconductor. Differentially expressed genes were identified using a twofold cutoff. GO terms enrichment was analysed using PANTHER ( http://www.pantherdb.org/ ) [33] or GOrilla ( http://cbl-gorilla.cs.technion.ac.il/ ) [34] . GSEA [35] was performed as described previously [36] . Gene expression fold changes in experimental cells relative to control were calculated and genes having at least twofold changes in shFOXA1-treated cells were defined as FOXA1-regulated gene sets. Differential expressed genes (at least twofold changes) in LNCaP shCtrl cells androgen-treated compared with hormone-deprived were defined as androgen-regulated gene sets. Raw and normalized data from microarray experiments have been deposited at NCBI Gene Expression Omnibus database (under accession GSE37314 and GSE55007 ). Cell proliferation assay Cell proliferation assay was carried out using the WST-1 kit according to the manufacturer’s instruction (Clontech). Briefly, cells were seeded in a 24-well plate at a density of 10,000 cells in 500 ul of complete culture medium and cultured in a CO 2 incubator at 37 °C for 24 h. Then cells were hormone starved for 2 to 3 days prior to WST-1 assay. Cultures were incubated for 2 h after the addition of the premixed WST-1 cell proliferation reagent and the absorbance at 450 nm was measured using a multiwell plate reader. The absorbance level of samples was normalized to that of the background control well (containing culture medium plus WST-1 reagent, without cells). Accession codes : New high-throughput sequence and microarray data generated in this study have been deposited in GEO database under accession code GSE55007 . How to cite this article : Jin, H.-J. et al. Cooperativity and equilibrium with FOXA1 define the androgen receptor transcriptional programme. Nat. Commun. 5:3972 doi: 10.1038/ncomms4972 (2014).